Ets2-dependent trophoblast signalling is required for gastrulation progression after primitive streak initiation Although extraembryonic ectoderm trophoblast signals the embryo for primitive streak initiation, a prerequisite for gastrulation, it is unknown whether it also signals for the progression of gastrulation after primitive streak initiation. Here, using Ets2−/− mice, we show that trophoblast signalling is also required in vivo for primitive streak elongation, completion of intraembryonic mesoderm epithelial–mesenchymal transition and the development of anterior primitive streak derivatives such as the node. We show that Ets2-dependent trophoblast signalling is required for the maintenance of high levels of Nodal and Wnt3 expression in the epiblast and for the induction of Snail expression in the primitive streak, between embryonic day 6.3 and 6.7. Within extraembryonic ectoderm trophoblast, Ets2 maintains the expression of the transcription factors Elf5, Cdx2 and Eomes , and that of the signalling molecule Bmp4. We propose a model that provides a genetic explanation as to how Ets2 in trophoblast mediates the progression of gastrulation within the epiblast. Gastrulation, a prerequisite for organogenesis, begins with the formation of the primitive streak (PS), where epiblast cells experience an epithelial-to-mesenchymal transition (EMT) to exit the epiblast and form the mesoderm and definitive endoderm (DE) layers. In mice, the PS appears around embryonic day 6.5 (E6.5) at the posterior end of the epiblast and elongates anteriorly. Mammalian gastrulation requires signals from two extraembryonic tissues: the visceral endoderm (VE—progenitor of yolk-sac endoderm and minor contributor to DE) and the extraembryonic ectoderm (EXE) trophoblast (progenitor of placental trophoblast) [1] , [2] . Although EXE trophoblast signalling is required for gastrulation initiation [3] , [4] , [5] , [6] , it is currently unknown whether it also controls gastrulation progression after PS initiation. This issue was addressed here using Ets2 homozygous null ( Ets2 −/−) mice. The transcription factor Ets2 is specifically expressed in EXE trophoblast, but not VE, before and during early gastrulation. Ets2−/− conceptuses die around E9.5 (refs 4 , 7 ) and display two main phenotypes: type-I and type-II ( [4] ). Both Ets2 −/− phenotypes represent an excellent in vivo system for investigating Ets2-mediated trophoblastic influcences on early embryogenesis. This is because embryonic development proceeds normally in: (a) chimaeras generated by aggregation of Ets2 +/+ tetraploid (4 n ) embryos (whose cells colonize the trophoblast and VE) with Ets2 −/− embryonic stem (ES) cells (which colonize the epiblast), (b) Ets2 −/− conceptuses on lentivirus-mediated trophoblast-specific Ets2 expression [7] , [8] . Ets2 −/− type-I mutants fail to initiate gastrulation and their distal VE (DVE) fails to become anterior VE (AVE—a sub-region of VE that patterns the epiblast) [4] . In contrast, Ets2 −/− type-II mutants form PS and AVE by the early PS stage [4] . However, it is unknown whether gastrulation can progress further in these mutants and their trophoblast phenotype is largely unexplored. We addressed these issues by examining gastrulation and trophoblast development in Ets2 −/− type-II mutants. We show that Ets2-dependent trophoblast signalling is required for gastrulation progression and controls processes including PS elongation, completion of mesoderm EMT and anterior PS derivative development. Evidence is provided about the timing of this trophoblast signalling. A genetic model is proposed to explain how trophoblast-derived Ets2 regulates gastrulation progression within the epiblast. Type-II versus type-I Ets2 −/− phenotypes As the crosses used here produced both Ets2 −/− phenotypes, it was important to be able to distinguish between them. During pregastrulation stages (E6.3), type-I mutants lack EXE character (loss of Bmp4 and Elf5 expression), show defective posterior epiblast (absence of Wnt3 expression) and exhibit an abnormally thickened DVE ( Fig. 1a ), consistent with previous findings [4] . During gastrulation (E6.7 and E7.5–7.75 stages) this DVE defect (that is, thickened VE region confined, entirely or partly, below the imaginary line that marks the luminal surface of distal tip epiblast) persists in type-I mutants (that is, mutants without a PS), as it was detected in mutants lacking Bra expression (PS marker) [4] or in those without any morphological signs of PS initiation on sectioning ( Fig. 1c ). This reflects their previously shown failure to form AVE [4] , confirmed here by Hex expression (DVE/AVE marker) [4] ( Fig. 1e ). In contrast, type-II mutants (that is, mutants with a PS, based on the presence of Bra or Cripto expression or morphological signs of PS in sections) never show such DVE thickening from at least E6.7 and up to E8.75 ( Figs 2b , 3a , 4d , 5c–f and 6d ). This is because they form an AVE by E6.7, as demonstrated by the expression pattern of the DVE/AVE markers Hex and Cer1 ( Fig. 6a–c ). These results show that during gastrulation, one can distinguish type-II from type-I mutants based on morphology (for example, no DVE thickening in type-II mutants) or PS marker gene expression (for example, Bra expression in type-II mutants). 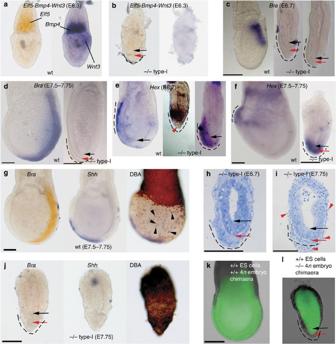Figure 1:  Unique aspects of theEts2type-I phenotype that distinguish it from that of type-II. (a,b) Double-colourin situhybridization for the expression ofElf5(orange),Bmp4(blue) andWnt3(blue) at E6.3 in controls (a) and type-I mutants (b). No expression is seen in the mutants. (c,d)Braexpression and gross morphology of type-I mutants and controls at E6.7 (c) and E7.5–7.75. (d) Note the absence ofBraexpression and a DVE thickening, which always includes a region below the level of the luminal surface of distal tip epiblast. (e,f)Hexexpression in controls and type-I mutants at E6.7 (e) and E7.5–7.75 (f). Note thatHexpositivity extends below the level of the luminal surface of distal tip epiblast. (g,j) Doublein situhybridization withBra(orange) andShh(blue), followed by DBA staining (brown) of the same embryo in E7.5–7.75 controls (g) and E7.75 type-I mutants (j). Note that type-I mutants (that is, mutants withoutBraexpression) do not expressShhand display continuous DBA positivity, indicative of failure to form DE. (h,i) Sagittal semithin sections of type-I mutants at E6.7 (h) and E7.75 (i), showing the DVE thickening and the absence of mesoderm or a PS. (k,l) E7.5–7.75 chimaeric embryos generated by aggregation of GFP-positiveEts2+/+ ES cells with GFP-negative tetraploid (4n) embryos, which are eitherEts2+/+ (k) orEts2−/− (l). Note that in contrast to controls, GFP positivity in type-I mutant chimaeras (that is, chimaeras with DVE thickening) does not extend to the outermost layer, indicating absence of DE. The posterior side in all embryos is on the right hand side. Black and red arrows depict the luminal side and outer side of distal tip epiblast, respectively. Dotted lines depict the localization of DVE/AVE along the anterior-posterior axis. Black arrowheads depict VE cells that experienced spreading, while red arrowheads depict regions of Richert’s membrane left attached to the embryo. Scale bars, 100 μm. Panelsa–candeandkandlare of the same magnification. Figure 1:  Unique aspects of the Ets2 type-I phenotype that distinguish it from that of type-II. ( a , b ) Double-colour in situ hybridization for the expression of Elf5 (orange), Bmp4 (blue) and Wnt3 (blue) at E6.3 in controls ( a ) and type-I mutants ( b ). No expression is seen in the mutants. ( c , d ) Bra expression and gross morphology of type-I mutants and controls at E6.7 ( c ) and E7.5–7.75. ( d ) Note the absence of Bra expression and a DVE thickening, which always includes a region below the level of the luminal surface of distal tip epiblast. ( e , f ) Hex expression in controls and type-I mutants at E6.7 ( e ) and E7.5–7.75 ( f ). Note that Hex positivity extends below the level of the luminal surface of distal tip epiblast. ( g , j ) Double in situ hybridization with Bra (orange) and Shh (blue), followed by DBA staining (brown) of the same embryo in E7.5–7.75 controls ( g ) and E7.75 type-I mutants ( j ). Note that type-I mutants (that is, mutants without Bra expression) do not express Shh and display continuous DBA positivity, indicative of failure to form DE. ( h , i ) Sagittal semithin sections of type-I mutants at E6.7 ( h ) and E7.75 ( i ), showing the DVE thickening and the absence of mesoderm or a PS. ( k , l ) E7.5–7.75 chimaeric embryos generated by aggregation of GFP-positive Ets2 +/+ ES cells with GFP-negative tetraploid (4 n ) embryos, which are either Ets2 +/+ ( k ) or Ets2 −/− ( l ). Note that in contrast to controls, GFP positivity in type-I mutant chimaeras (that is, chimaeras with DVE thickening) does not extend to the outermost layer, indicating absence of DE. The posterior side in all embryos is on the right hand side. Black and red arrows depict the luminal side and outer side of distal tip epiblast, respectively. Dotted lines depict the localization of DVE/AVE along the anterior-posterior axis. Black arrowheads depict VE cells that experienced spreading, while red arrowheads depict regions of Richert’s membrane left attached to the embryo. Scale bars, 100 μm. Panels a–c and e and k and l are of the same magnification. 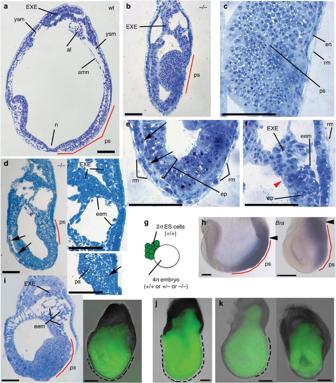Figure 2:  Defective gastrulation progression inEts2type-II mutants and type-II mutant chimaeras. (a–f) Sagittal semithin sections of E7.75 wild-type (a) and type-II mutants at E7.75 (b) and E8.75 (d). Panelsc,eandfare magnifications of the PS, distal tip and embryonic–extraembryonic junction regions inb, respectively, and bottom-right image in paneldare high magnifications of the PS region ofbandd, respectively. Top-right and bottom-right images indare magnifications of the extraembryonic and PS regions shown in left image ofd, respectively. Note the abnormal cellular accumulation at the PS, absence of intraembryonic mesenchymal cells (b–d), oval cells adjacent to the epiblast (arrows ineandd), extraembryonic mesoderm (probably yolk-sac mesoderm infandd) and lack of morphologically recognizable amnion, allantois, node (b,d). (g) Schematic of the protocol used to generateEts2type-II mutant chimaeras: aggregation of GFP-expressingEts2+/+ ES cells with a non-GFP-expressing tetraploid embryo (genotype was eitherEts2+/+,Ets2+/−, orEts2−/−). (h)Braexpression in E7.75 control (tetraploid embryoEts2+/+or −/+; left panel) and mutant (tetraploid embryoEts2−/−;right panel) chimaeras. (i) Sagittal semithin section (left image) and whole-mount GFP fluorescent view (right image) of the same E7.75 type-II mutant chimaera. Note its morphological resemblance to its non-chimaeric type-II mutant counterparts. (j,k) Whole-mount GFP fluorescent views of E7.75 control chimaera (j) and two E7.75 type-II mutant chimaeras (k). Note that the VE in the majority of these mutant chimaeras (4/6), contains GFP positivity (dotted lines ini–k) albeit to a lesser extent than that of controls (j). The VE in the rest of these chimaeras however (2/6), is GFP-negative. In all panels posterior is to the right, red lines denote apparent PS length. Arrowheads infandhdepict the embryonic–extraembryonic junction. Scale bars, 10 μm (a–f,h,i(left image)), 20 μm (i(right image),j,k). al, allantois; amn, amnion; eem, extraembryonic mesoderm; en, endoderm; ep, epiblast; n, node; ps, primitive streak; rm, Richert’s membrane, ysm, yolk-sac mesoderm. Full size image Figure 2:  Defective gastrulation progression in Ets2 type-II mutants and type-II mutant chimaeras. ( a–f ) Sagittal semithin sections of E7.75 wild-type ( a ) and type-II mutants at E7.75 ( b ) and E8.75 ( d ). Panels c , e and f are magnifications of the PS, distal tip and embryonic–extraembryonic junction regions in b , respectively, and bottom-right image in panel d are high magnifications of the PS region of b and d , respectively. Top-right and bottom-right images in d are magnifications of the extraembryonic and PS regions shown in left image of d , respectively. Note the abnormal cellular accumulation at the PS, absence of intraembryonic mesenchymal cells ( b – d ), oval cells adjacent to the epiblast (arrows in e and d ), extraembryonic mesoderm (probably yolk-sac mesoderm in f and d ) and lack of morphologically recognizable amnion, allantois, node ( b , d ). ( g ) Schematic of the protocol used to generate Ets2 type-II mutant chimaeras: aggregation of GFP-expressing Ets2 +/+ ES cells with a non-GFP-expressing tetraploid embryo (genotype was either Ets2 +/+, Ets2 +/−, or Ets2 −/−). ( h ) Bra expression in E7.75 control (tetraploid embryo Ets2+/+ or −/+; left panel) and mutant (tetraploid embryo Ets2−/−; right panel) chimaeras. ( i ) Sagittal semithin section (left image) and whole-mount GFP fluorescent view (right image) of the same E7.75 type-II mutant chimaera. Note its morphological resemblance to its non-chimaeric type-II mutant counterparts. ( j , k ) Whole-mount GFP fluorescent views of E7.75 control chimaera ( j ) and two E7.75 type-II mutant chimaeras ( k ). Note that the VE in the majority of these mutant chimaeras (4/6), contains GFP positivity (dotted lines in i – k ) albeit to a lesser extent than that of controls ( j ). The VE in the rest of these chimaeras however (2/6), is GFP-negative. In all panels posterior is to the right, red lines denote apparent PS length. Arrowheads in f and h depict the embryonic–extraembryonic junction. Scale bars, 10 μm ( a–f , h , i (left image)), 20 μm ( i (right image), j , k ). al, allantois; amn, amnion; eem, extraembryonic mesoderm; en, endoderm; ep, epiblast; n, node; ps, primitive streak; rm, Richert’s membrane, ysm, yolk-sac mesoderm. 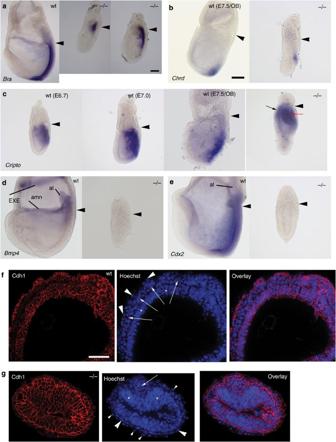Figure 3:Ets2type-II mutants display defective PS development. (a,b)BraandChrdexpression at E7.5 in control (left panels inaandb) and mutant embryos (right panels inaandb), showing failure of PS elongation. (c)Criptoexpression (PS and intraembryonic mesoderm marker) in control embryos at E6.7, E7.0 and E7.5 (first three panels from the left) and in an E7.5 mutant (fourth panel from the left), which expresses it in the PS and mesoderm (red arrow) and ectopically in the proximal-anterior epiblast (black arrow). (d)Bmp4expression at E7.5–7.75 (allantois, amnion, EXE and posterior PS marker) in control (left panel) and a mutant (right panel) embryo that shows no expression. (e)Cdx2at E7.5–7.75 (allantois, PS and EXE marker) is expressed in controls (left panel and data not shown), but not in the mutant (right panel). (f,g) Fluorescent views of sections perpendicular to the long axis of the embryo at the level of the PS at E7.75 from control (depicted inf) and mutant embryo (depicted ing), showing E-cadherin (Cdh1) protein localization (red fluorescence) and nuclei (blue fluorescence). In controls, Cdh1 positivity marks the epiblast (asterisks inf) and the outermost layer (endoderm; white arrowheads inf), but not the epiblast-derived mesoderm cells (white arrows inf). In the mutant, although Cdh1 positivity also marks the epiblast and endoderm (asterisks and large white arrowheads ing, respectively), it fails to become downregulated from the mesoderm (white arrow ing). Note that cells of Richert’s membrane (normally Cdh1 negative) are present in the mutant (small arrowheads ing), because they were not removed. Black arrowheads depict the embryonic–extraembryonic junction at the posterior side of the embryo. All embryos ina–ewere subjected to whole-mountin situhybridization. All embryos inaare of the same magnification, as are those inb–e. All sections infandgare of the same magnification. Scale bars, 10 μm (a,b), 5 μm (f). al, allantois; amn, amnion; OB, no allantoic bud stage. Full size image Figure 3: Ets2 type-II mutants display defective PS development. ( a , b ) Bra and Chrd expression at E7.5 in control (left panels in a and b ) and mutant embryos (right panels in a and b ), showing failure of PS elongation. ( c ) Cripto expression (PS and intraembryonic mesoderm marker) in control embryos at E6.7, E7.0 and E7.5 (first three panels from the left) and in an E7.5 mutant (fourth panel from the left), which expresses it in the PS and mesoderm (red arrow) and ectopically in the proximal-anterior epiblast (black arrow). ( d ) Bmp4 expression at E7.5–7.75 (allantois, amnion, EXE and posterior PS marker) in control (left panel) and a mutant (right panel) embryo that shows no expression. ( e ) Cdx2 at E7.5–7.75 (allantois, PS and EXE marker) is expressed in controls (left panel and data not shown), but not in the mutant (right panel). ( f , g ) Fluorescent views of sections perpendicular to the long axis of the embryo at the level of the PS at E7.75 from control (depicted in f ) and mutant embryo (depicted in g ), showing E-cadherin (Cdh1) protein localization (red fluorescence) and nuclei (blue fluorescence). In controls, Cdh1 positivity marks the epiblast (asterisks in f ) and the outermost layer (endoderm; white arrowheads in f ), but not the epiblast-derived mesoderm cells (white arrows in f ). In the mutant, although Cdh1 positivity also marks the epiblast and endoderm (asterisks and large white arrowheads in g , respectively), it fails to become downregulated from the mesoderm (white arrow in g ). Note that cells of Richert’s membrane (normally Cdh1 negative) are present in the mutant (small arrowheads in g ), because they were not removed. Black arrowheads depict the embryonic–extraembryonic junction at the posterior side of the embryo. All embryos in a – e were subjected to whole-mount in situ hybridization. All embryos in a are of the same magnification, as are those in b–e . All sections in f and g are of the same magnification. Scale bars, 10 μm ( a , b ), 5 μm ( f ). al, allantois; amn, amnion; OB, no allantoic bud stage. 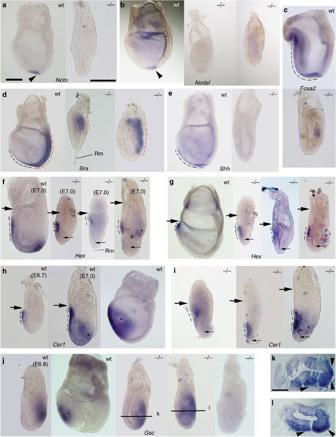Figure 4:  Marker gene expression inEts2type-II mutants. (a,b) Absence of node markersNotoandNodal(arrowheads in controls) from E7.5-E7.75 mutants. (c–e) Absence of anterior and distal expression ofFoxa2(node and AME marker; dotted lines inc),Bra(PS and node/head process marker; black and red dotted lines ind, respectively) andShh(node and AME marker; dotted lines ine) in E7.75 mutants. (f,g)Hexexpression (AVE and anterior DE marker, dotted lines and asterisk, respectively) in E7.0 (f) and E7.5–7.75 (g) mutants. Note that some, but not all, mutants possess DE, while some fail to completely anteriorize AVE localization. (h,i)Cer1expression (AVE and anterior DE marker; dotted lines and asterisk, respectively) in controls at E6.7, E7.0 and E7.75 (h) and in E7.75 mutants (g). Note that in some mutants DE forms and that AVE localization fails to anteriorize completely. (j)Gscexpression (anterior PS and anterior DE marker, the latter depicted by an asterisk) in controls at E6.8 and at E7.5–7.75 (first and second panels from the left, respectively) and in E7.5-E7.75 mutants (last three left hand side images). Note that some mutants show DE formation. (k,l) Cross-sections of the mutants shown inj(third and fourth images from the left, respectively), taken from where the black lines are, showing expression in the anterior epiblast and in the posterio-lateral outermost layer (DE cells), indicated by arrowheads. All panels exceptkandlshow whole-mountin situhybridizations, with the posterior embryo side being on the right. Large and small arrows depict the embryonic–extraembryonic junction and the luminal surface of distal tip epiblast, respectively. Asterisks mark DE cells. All whole-mount control (wt) embryos are of the same magnification, as are all mutant ones. Rm, Richert’s membrane. Scale bar, 20 μm (a(control)), 20 μm (a(mutant)). Sections inkandlare of the same magnification. Scale bar, 50 μm (k). Full size image Figure 4:  Marker gene expression in Ets2 type-II mutants. ( a , b ) Absence of node markers Noto and Nodal (arrowheads in controls) from E7.5-E7.75 mutants. ( c – e ) Absence of anterior and distal expression of Foxa2 (node and AME marker; dotted lines in c ), Bra (PS and node/head process marker; black and red dotted lines in d , respectively) and Shh (node and AME marker; dotted lines in e ) in E7.75 mutants. ( f , g ) Hex expression (AVE and anterior DE marker, dotted lines and asterisk, respectively) in E7.0 ( f ) and E7.5–7.75 ( g ) mutants. Note that some, but not all, mutants possess DE, while some fail to completely anteriorize AVE localization. ( h , i ) Cer1 expression (AVE and anterior DE marker; dotted lines and asterisk, respectively) in controls at E6.7, E7.0 and E7.75 ( h ) and in E7.75 mutants ( g ). Note that in some mutants DE forms and that AVE localization fails to anteriorize completely. ( j ) Gsc expression (anterior PS and anterior DE marker, the latter depicted by an asterisk) in controls at E6.8 and at E7.5–7.75 (first and second panels from the left, respectively) and in E7.5-E7.75 mutants (last three left hand side images). Note that some mutants show DE formation. ( k , l ) Cross-sections of the mutants shown in j (third and fourth images from the left, respectively), taken from where the black lines are, showing expression in the anterior epiblast and in the posterio-lateral outermost layer (DE cells), indicated by arrowheads. All panels except k and l show whole-mount in situ hybridizations, with the posterior embryo side being on the right. Large and small arrows depict the embryonic–extraembryonic junction and the luminal surface of distal tip epiblast, respectively. Asterisks mark DE cells. All whole-mount control (wt) embryos are of the same magnification, as are all mutant ones. Rm, Richert’s membrane. Scale bar, 20 μm ( a (control)), 20 μm ( a (mutant)). Sections in k and l are of the same magnification. Scale bar, 50 μm ( k ). 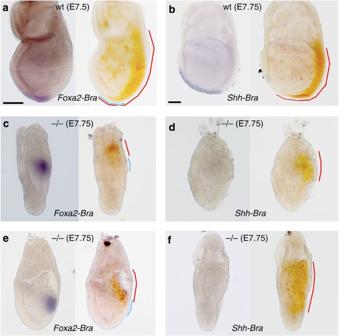Figure 5:  Node and AME development inEts2type-II mutants. (a,c,e) Double-colourin situhybridization withFoxa2(blue) andBra(orange) in control E7.5 embryos (a) and E7.75 mutants (cande). In controls, the node is a region at the distal tip of the embryo that can be defined by the complete overlap betweenFoxa2andBraexpression (overlap between blue and red lines ina). In the mutants, there is no distalFoxa2orBraexpression or any significant overlap between their expression patterns, irrespective of whether the PS is only about 1/5th (c) or about half the proximo-distal length of the posterior epiblast (e). (b,d,f) Double-colourin situhybridization withShh(a marker of the node and AME; blue signal) andBra(yellow/orange signal) in wild-type E7.75 embryos (b) and E7.75 type-II mutants (d,f). Note the absence ofShhexpression in mutants with short (d) or longer (f) PS. The posterior side in all embryos is on the right hand side. In all the panels, each pair of images is of the same embryo, with the left image (Foxa2orShh) photographed last, after alcohol-mediated disappearance ofBraexpression and completion ofFoxa2/Shhcolour detection procedures. Red and blue lines represent the anterior-posterior extent ofBraandFoxa2expression, respectively. Panelsaandc–fare of the same magnification; Scale bar, 100 μm (a,b). Full size image Figure 5:  Node and AME development in Ets2 type-II mutants. ( a , c , e ) Double-colour in situ hybridization with Foxa2 (blue) and Bra (orange) in control E7.5 embryos ( a ) and E7.75 mutants ( c and e ). In controls, the node is a region at the distal tip of the embryo that can be defined by the complete overlap between Foxa2 and Bra expression (overlap between blue and red lines in a ). In the mutants, there is no distal Foxa2 or Bra expression or any significant overlap between their expression patterns, irrespective of whether the PS is only about 1/5th ( c ) or about half the proximo-distal length of the posterior epiblast ( e ). ( b , d , f ) Double-colour in situ hybridization with Shh (a marker of the node and AME; blue signal) and Bra (yellow/orange signal) in wild-type E7.75 embryos ( b ) and E7.75 type-II mutants ( d , f ). Note the absence of Shh expression in mutants with short ( d ) or longer ( f ) PS. The posterior side in all embryos is on the right hand side. In all the panels, each pair of images is of the same embryo, with the left image ( Foxa2 or Shh ) photographed last, after alcohol-mediated disappearance of Bra expression and completion of Foxa2/Shh colour detection procedures. Red and blue lines represent the anterior-posterior extent of Bra and Foxa2 expression, respectively. Panels a and c–f are of the same magnification; Scale bar, 100 μm ( a , b ). 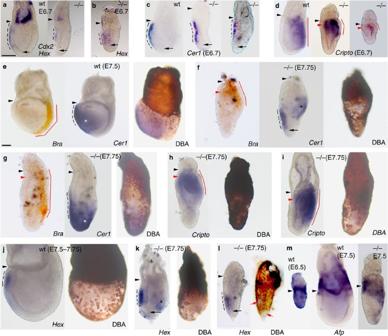Figure 6:  Marker gene expression and DBA staining inEts2type-II mutants. (a–c) Expression ofHex/Cdx2: simultaneous detection of both (a), onlyHex(b) and onlyCer1(c) at E6.7. Note the failure of AVE (Hex/Cer1positivity) to closely approach the anterior embryonic–extraembryonic junction in most mutants. (d)Criptoexpression in E6.7 mutants showing a short PS in all and ectopic expression in anterior epiblast in some. (e–g) Double-colourin situhybridization withBra(orange) andCer1(blue), followed by DBA staining (brown) of the same embryo in E7.5-E7.75 controls (e) and two E7.75 type-II mutants (f,g). Mutants can fail to completely anteriorize their AVE (AVE expression ofCer1infandg) and can form DE (non-AVE expression ofCer1; asterisks infandgand patchy DBA positivity infandg). When AVE fails to reach the anterior 40% of anterior epiblast, there is ectopic expression ofBrain anterior epiblast (f) and when it doesn’tBraexpression remains posterior (g). (h,i) E7.75 mutants showingCriptoexpression and DBA staining: some do not form DE (continuous DBA positivity inh), while others do (patchy DBA staining ini). (j–i) E7.5–7.75 wild (j) and E7.75 mutants (k,l) showingHexexpression and DBA staining: patchy DBA staining (right image inkand red arrows in right image ofl) was associated with the presence (asterisk ink) or absence (left image inl) of non-AVEHexexpression. (m)Afpexpression in wild E6.5 and E7.5 (left and middle images, respectively) and E7.5 type-II mutant (right image). In all, posterior is to the right. Black and red arrowheads depict the anterior embryonic–extraembryonic junction and proximo-anterior epiblast, respectively. Arrows mark the luminal side of distal tip epiblast. Dotted lines mark the antero-posterior extent of AVE, red lines that of the PS and asterisks the DE. All images in panelsa–dandf–mexcept middle image inmare of the same magnification. Scale bar, 100 μm (a). Paneleand middle image in panelmare of the same magnification; scale bar, 100 μm (e). Full size image Figure 6:  Marker gene expression and DBA staining in Ets2 type-II mutants. ( a–c ) Expression of Hex / Cdx2 : simultaneous detection of both ( a ), only Hex ( b ) and only Cer1 ( c ) at E6.7. Note the failure of AVE ( Hex / Cer1 positivity) to closely approach the anterior embryonic–extraembryonic junction in most mutants. ( d ) Cripto expression in E6.7 mutants showing a short PS in all and ectopic expression in anterior epiblast in some. ( e–g ) Double-colour in situ hybridization with Bra (orange) and Cer1 (blue), followed by DBA staining (brown) of the same embryo in E7.5-E7.75 controls ( e ) and two E7.75 type-II mutants ( f , g ). Mutants can fail to completely anteriorize their AVE (AVE expression of Cer1 in f and g ) and can form DE (non-AVE expression of Cer1 ; asterisks in f and g and patchy DBA positivity in f and g ). When AVE fails to reach the anterior 40% of anterior epiblast, there is ectopic expression of Bra in anterior epiblast ( f ) and when it doesn’t Bra expression remains posterior ( g ). ( h , i ) E7.75 mutants showing Cripto expression and DBA staining: some do not form DE (continuous DBA positivity in h ), while others do (patchy DBA staining in i ). ( j–i ) E7.5–7.75 wild ( j ) and E7.75 mutants ( k , l ) showing Hex expression and DBA staining: patchy DBA staining (right image in k and red arrows in right image of l ) was associated with the presence (asterisk in k ) or absence (left image in l ) of non-AVE Hex expression. ( m ) Afp expression in wild E6.5 and E7.5 (left and middle images, respectively) and E7.5 type-II mutant (right image). In all, posterior is to the right. Black and red arrowheads depict the anterior embryonic–extraembryonic junction and proximo-anterior epiblast, respectively. Arrows mark the luminal side of distal tip epiblast. Dotted lines mark the antero-posterior extent of AVE, red lines that of the PS and asterisks the DE. All images in panels a–d and f–m except middle image in m are of the same magnification. Scale bar, 100 μm ( a ). Panel e and middle image in panel m are of the same magnification; scale bar, 100 μm ( e ). Full size image In addition to being devoid of PS and mesoderm [4] , type-I mutants (that is, mutants that lack Bra expression) also lack DE and probably node and anterior axial mesendoderm (AME) by E7.5–7.75. This was based on: (a) absence of Shh expression (marker of node and AME [9] ) and (b) absence of patchy DBA lectin positivity within the epiblast-associated VE ( Fig. 1g ). Although DBA lectin specifically stains all VE, but not DE, mesoderm or epiblast cells [10] , [11] , it can be used as an indirect marker of DE formation. This is because during normal development, when DE cells intercalate into the epiblast-associated VE to form the DE layer, the initially closely packed VE cells (continuous DBA positivity) become dispersed in this part of the VE (patchy DBA positivity) to accommodate the newly formed DE cells, whereas this VE dispersal does not occur in the EXE-associated VE, where DE does not form (continuous DBA positivity) [12] ( Fig. 1g , right panel). The absence of DE and presence of DVE thickening in type-I mutants was also seen in a subset of E7.5–7.75 aggregation chimaeras made with Ets2 +/+/GFP-positive ES cells and an Ets2 −/− 4 n /GFP-negative embryo, the so-called ‘type-I chimaeras’. This is shown by the absence of GFP positivity in their VE, which is thickened distally ( Fig. 1k ). These results are consistent with previous examination of type-I chimaeras [4] and confirm that Ets2 in trophoblast is also required for PS derivative formation such as the DE, in the context of type-I phenotype. Failure of gastrulation progression in type-II mutants Semithin sagittal sections of E7.75 type-II mutants (henceforth also referred to as ‘mutants’) showed several gastrulation defects. First, we observed cell accumulation at the PS and absence of intraembryonic mesenchymal cells anteriorly ( n =2; Fig. 2b ), suggesting failure of PS to elongate and intraembryonic mesoderm to migrate away from the PS. Second, the absence of any recognizable allantois or amnion and the limited extraembryonic mesoderm (putative yolk-sac mesoderm) formation in these mutants ( n =2; Fig. 2b ) indicates defective development of posterior and proximal epiblast derivatives. Third, an anatomical node (anterior PS derivative), which at E7.5–7.75 constitutes a bilayered structure at the distal tip of the embryo [13] , [14] ( Fig. 2a ), was never observed in the mutants ( n =2; Fig. 2b ). Fourth, oval-to-flattened cells situated between the epiblast and the outermost endodermal layer, were observed in the mutants ( n =2; Fig. 2e ), but not controls ( Fig. 2a ). This may signify DE formation in at least some of the mutants because the shape of these cells resembles that of DE cells in E7.0 wild-type embryos, just before they intercalate within the VE [14] . Inspection of sections from mutants at E8.75 (that is, just before their death) revealed a similar phenotype ( n =2; Fig. 2d ). Ets2 in trophoblast is required for gastrulation progression To confirm that lack of Ets2 in trophoblast is responsible for the type-II phenotype, we generated chimaeras by aggregating GFP-positive Ets2 +/+ ES cells with GFP-negative 4 n embryos (either Ets2 −/−, −/+, or +/+) ( Fig. 2g ). When the tetraploid embryo used was Ets2 −/−, inspection at E7.75 showed that these ‘mutant’ chimaeras either phenocopied the type-I phenotype [4] ( Fig. 1i ) or that of type-II ( Fig. 2h ). In the latter case, all major morphological aspects of type-II mutants were found in these ‘type-II chimaeras’. These included: (a) A short PS based on Bra expression ( n =2; Fig. 2h ) and morphology ( n =2; Fig. 2i) . (b) Defective intraembryonic mesoderm development evidenced by a cellular accumulation in the PS region and absence of anterior intraembryonic mesenchymal cells ( n =2; Fig. 2i ). (c) Absence of a morphologically identifiable node, allantois and amnion and limited extraembryonic mesoderm formation ( n =2; Fig. 2i ). GFP positivity in control chimaeras (4 n embryo used was either Ets2 +/+ or +/−) reached the epiblast-associated VE layer throughout its anterior-posterior (A-P) extent ( Fig. 2j ), indicative of DE formation [12] . In type-II chimaeras however, GFP positivity reached the epiblast-associated VE in most cases ( n =4/6), but this was not evident throughout the A-P axis of VE ( Fig. 2i ), while in the remaining minority ( n =2/6), no GFP signal was seen in the VE ( Fig. 2k ). One interpretation of these chimaera results is that in the majority of type-II mutants, DE forms at reduced levels and in a minority it does not (see below). Defective PS and mesoderm development in type-II mutants The aforementioned shortness of the mutant PS was confirmed by the expression patterns of Bra (ref. 4 ) ( n =3) and the anterior PS marker Chrd (ref. 15 ) ( n =3) in E7.5 mutants ( Fig. 3a ). Cripto , a marker of PS and intraembryonic mesoderm up to E7.0 that becomes confined to the PS by E7.5 ( [16] ), was expressed in the PS region of E7.5 mutants ( n =3; Fig. 3c ), confirming that the aforementioned cell accumulation at the mutant PS represents specified mesoderm. The above-mentioned absence of anatomical allantois and amnion in the mutants was confirmed by the lack of embryonic expression of Bmp4 and Cdx2 in E7.5 mutants ( n =3; Fig. 3d ), both of which normally mark the base of allantois, with Bmp4 also marking the amnion [17] , [18] , [19] ( Fig. 3d ). Normally, Bmp4 and Cdx2 expression patterns at E7.5 also mark the posterior PS or the entire PS, respectively [17] , [18] , [19] , but are absent in these regions in the mutants ( n =3; Fig. 3d ), suggesting defective A-P patterning of the PS. The aforementioned failure of intraembryonic mesoderm to migrate away from the mutant PS is due to failure of mesoderm cells to complete their EMT. Although epiblast cells in the PS of E7.75 mutants lose their elongated (epithelial) shape ( Figs 2c and 3g ), a process indicative of EMT initiation, they fail to also downregulate the levels of Cdh1 (E-cadherin) protein ( n =2; Fig. 3f ), a marker of the epithelial epiblast and VE cells, but not of the mesenchymal PS-derived mesoderm cells [20] . Anterior PS derivative development in type-II mutants To investigate in more detail the development of anterior PS derivatives (node, AME and DE) [13] , [21] in the mutants, we first examined the expression of the node markers Noto and Nodal [22] , [23] at E7.5–7.75. We found that Noto is not expressed ( n =4/4; Fig. 4a ) and Nodal expression was either absent ( n =2/4), or barely detectable ( n =2/4) in the PS region ( Fig. 4b ), indicating failure of node cell specification. The AME, an axial structure anterior to the node [13] , is incorrectly specified and may be absent from E7.75 mutants. This was based on absence from the anterior half of the embryo of the expression of Bra (marker of entire PS, node and posterior AME by E7.75; [24] ) ( n =3; Fig. 4d ), as well as that of Foxa2 ( n =4) and Shh ( n =3) (markers of node and entire AME by E7.75; [9] , [13] ; Fig. 4c ). We confirmed that these defects are part of the type-II phenotype (that is, mutants expressing Bra ) and independent of any variability in the developmental stage (based on PS length of the mutants). Simultaneous examination of Bra - Foxa2 expression in E7.5 mutants (for node specification, defined as a distal tip region co-expressing Bra and Foxa2; [13] , [24] ) or that of Bra-Shh in E7.75 mutants (for AME specification), revealed absence of Bra-Foxa2 co-expression at the distal tip ( n =4; Fig. 5a ) and non-appearance of Shh expression ( n =4; Fig. 5b ), irrespective of PS length (based on A-P length of Bra positivity). We next investigated the expression of Hex and Cer1 , both of which mark the AVE at all stages and the DE when it first appears in the distal region of the embryo around E7.0, with Cer1 expression remaining in the anterior DE up to E7.5–7.75 ( Figs 4f–h and 6a ; [13] , [25] ). Although type-II mutants form an AVE, its anterior edge fails to closely approach the anterior embryonic–extraembryonic junction in most cases, as shown by the expression of Hex or Cer1 at E6.7 ( n =3/4; Fig. 6a–c ), Hex at E7.0 ( n =4/6; Fig. 4f ) and Hex ( n =8/9) or Cer1 ( n =9/11) at E7.75 ( Fig. 4g–i ). Confirmation that this AVE anteriorization defect belongs to the type-II phenotype and that it is unrelated to the developmental stage of the mutants, came from its detection in the majority ( n =3/4) of E7.75 mutants, all of which possessed a PS of variable lengths, on simultaneous examination of Bra and Cer1 expression in the same embryo ( Fig. 6e–g ). As AVE normally inhibits posterior epiblast character (for example,. Bra and Cripto expression) from anterior epiblast [26] , this AVE defect could explain the ectopic expression of these genes in the anterior epiblast in 37% ( n =7/19) of E7.75 type-II mutants ( Figs 3c , 4d and 6f ). This is consistent with 44% ( n =8/18) of E7.75 type-II mutants failing to translocate the anterior edge of their AVE into the anterior 40% of anterior epiblast, based on Hex and Cer1 expression patterns. The non-AVE (putative DE) expression patterns of Hex and Cer1 were detected in a minority of mutants at E7.0 ( n =1/6 for Hex ; Fig. 4f ) and in about half at E7.5–7.75 ( n =4/9 for Hex and n =6/11 for Cer1 ; Figs 4g–i and 6f ). However, absence of Hex/Cer1 expression in DE does not necessarily mean absence of DE because Hex−/− embryos form a DE that lacks Cer1 expression [27] . Importantly, DE formation was detected in most ( n =3/4) E7.5–7.75 type-II mutants based on whole-mount and cross-sectional views of Gsc expression ( Fig. 4j–l ), which normally marks anterior DE and anterior PS epiblast from around E7.0 and by E7.5–7.75 becomes restricted to the anterior AME [28] . To assess DE formation in its entirety and to confirm that any DE defects seen belong to the type-II phenotype (that is, mutants with a PS), we carried out DBA lectin staining (see above) in E7.75 mutants previously subjected to RNA in situ hybridization with the PS markers Bra or Cripto . We found that the majority ( n =12/14; 86%) of type-II mutants form DE, as judged by the presence of patchy DBA staining. However, patchy DBA staining was not evident in the most proximal epiblast-associated VE ( n =12/12), indicating reduced DE formation ( Fig. 6e–i ). This is consistent with: (a) Afp expression being confined to the proximal epiblast-associated VE of E7.5 mutants ( n =3; Fig. 6m ), as it normally marks the entire epiblast-associated VE and on DE formation becomes downregulated from VE cells that experience spreading to accommodate the DE [12] , [29] and (b) the limited GFP signal in the VE of type-II mutant chimaeras (see above). No correlation was found between PS length and DBA-based DE detection, as mutants with similar PS lengths may or may not display DE formation ( Fig. 6f ). Although non-AVE (that is, putative DE) Cer1/Hex expression in the mutants was always associated with patchy DBA positivity ( n =4/4; Fig. 6e–g ), such DBA staining was not always observed in mutants lacking non-AVE Cer1/Hex expression ( n =2/4; Fig. 6j ). This indicates that Hex/Cer1 expression-based DE detection underestimates the occurrence of DE formation and is consistent with the higher DE detection percentage based on Gsc expression or DBA staining. Regulatory gene expression in type-II mutant epiblast To investigate regulatory gene expression within the epiblast of type-II mutants (that is, mutants without DVE thickening), we first examined the expression of Nodal at E6.7, as high levels of epiblast Nodal expression/signalling are required for PS elongation and formation of anterior PS derivatives [9] , [30] , [31] . Nodal expression levels are reduced in E6.7 mutants, as judged by RNA in situ hybridization ( n =4/5; Fig. 7a ) and quantitative real-time PCR (qRT–PCR) ( n =4; Fig. 8 ). We next investigated the PS expression of the transcription factors Eomes and Snail , which are required in epiblast/PS for intraembryonic EMT [20] , [32] and that of the secreted molecule Fgf8 , which is required in the PS for mesoderm migration, rather than EMT [33] . Although Eomes PS expression was undetectable in E6.7 mutants ( n =3; Fig. 7b ), by E7.75 it was observed at levels similar to those in the PS of E6.7 control embryos, suggesting a delay in its onset of expression ( n =5; Fig. 7c ). In contrast, Snail expression was undetectable in the mutants at E6.7 ( n =3; Fig. 7d ) and barely detectable at E7.75 ( n =5; Fig. 7e ). Fgf8 expression on the other hand, was detectable in E6.7 mutants at apparently normal levels ( n =3; Fig. 7f ). 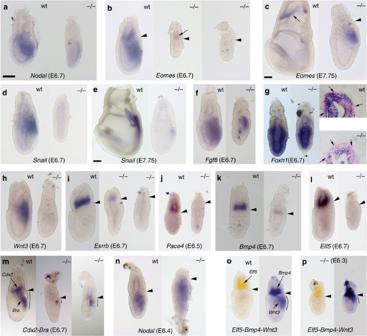Figure 7:  Regulatory gene expression in trophoblastic and embryonic regions inEts2type-II mutants. (a)Nodalexpression at E6.7 in controls (left) and mutants (right). Note the downregulation ofNodalin the mutants. (b,c)Eomesexpression at E6.7 (b) and E7.75 (c) in controls (left images) and mutants (middle and right images). (d,e)Snailis expressed in the PS of E6.7 and E7.75 controls (left images indande, respectively), but downregulated in the mutants (right images indande, respectively). (f)Fgf8is expressed at normal levels in the short PS of E6.7 mutants (right image). (g)Foxh1is expressed in epiblast of controls (left image) and mutants (middle image), but absent from the mutant VE, as confirmed in cross-sections (images on the right; arrows denote the VE layer). (h)Wnt3is expressed in the PS of controls (left), but not that of mutants (right). (i–l) EXE expression ofEsrrb(i),Pace4(j),Bmp4(k) andElf5(l) in controls (left images) and mutants (right images) at E6.7 or E6.5. In the mutants,Esrrbis either barely detectable or absent,Bmp4is greatly downregulated, whilePace4andElf5are undetectable. (m) Single-colourin situhybridization for the simultaneous detection ofCdx2andBraexpression in E6.7 controls (left image) and mutants (right images). AlthoughBrais expressed in the PS of controls and mutants,Cdx2is expressed in the EXE of controls, but is undetectable (middle image) or greatly reduced (right image) in the mutants. (n)Nodalexpression in E6.4 controls (left) and mutants (right). (o,p) Double-colourin situhybridization for the expression ofElf5(orange),Bmp4(blue) andWnt3(blue) in controls (o) and mutants (p) at E6.3. Both images in (o,p) are of the same embryo. All three genes are expressed similarly between controls and mutants. In all, posterior is to the right. Arrowheads depict the embryonic–extraembryonic junction and asterisks signify Richert’s membrane that was not removed. All embryos are of the same magnification, except the left images in panelscande. Scale bars, 10 μm. Figure 7:  Regulatory gene expression in trophoblastic and embryonic regions in Ets2 type-II mutants. ( a ) Nodal expression at E6.7 in controls (left) and mutants (right). Note the downregulation of Nodal in the mutants. ( b , c ) Eomes expression at E6.7 ( b ) and E7.75 ( c ) in controls (left images) and mutants (middle and right images). ( d , e ) Snail is expressed in the PS of E6.7 and E7.75 controls (left images in d and e , respectively), but downregulated in the mutants (right images in d and e , respectively). ( f ) Fgf8 is expressed at normal levels in the short PS of E6.7 mutants (right image). ( g ) Foxh1 is expressed in epiblast of controls (left image) and mutants (middle image), but absent from the mutant VE, as confirmed in cross-sections (images on the right; arrows denote the VE layer). ( h ) Wnt3 is expressed in the PS of controls (left), but not that of mutants (right). ( i – l ) EXE expression of Esrrb ( i ), Pace4 ( j ), Bmp4 ( k ) and Elf5 ( l ) in controls (left images) and mutants (right images) at E6.7 or E6.5. In the mutants, Esrrb is either barely detectable or absent, Bmp4 is greatly downregulated, while Pace4 and Elf5 are undetectable. ( m ) Single-colour in situ hybridization for the simultaneous detection of Cdx2 and Bra expression in E6.7 controls (left image) and mutants (right images). Although Bra is expressed in the PS of controls and mutants, Cdx2 is expressed in the EXE of controls, but is undetectable (middle image) or greatly reduced (right image) in the mutants. ( n ) Nodal expression in E6.4 controls (left) and mutants (right). ( o , p ) Double-colour in situ hybridization for the expression of Elf5 (orange), Bmp4 (blue) and Wnt3 (blue) in controls ( o ) and mutants ( p ) at E6.3. Both images in ( o , p ) are of the same embryo. All three genes are expressed similarly between controls and mutants. In all, posterior is to the right. Arrowheads depict the embryonic–extraembryonic junction and asterisks signify Richert’s membrane that was not removed. All embryos are of the same magnification, except the left images in panels c and e . Scale bars, 10 μm. 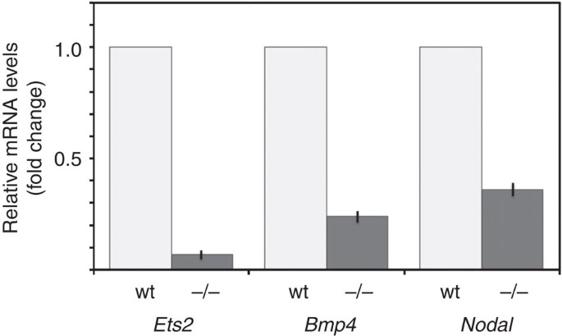Figure 8:  Real-time PCR (qRT–PCR) gene expression level quantification in E6.7Ets2type-II mutant embryos. Graph showing the mean values of fold change forEts2,Bmp4andNodalmRNA levels in E6.7 mutants (dark grey columns) relative to those of E6.7 wild-type (wt) control embryos (light-grey columns). Both control and mutant values were relative to those of the internal control genebeta-actin, with mutant values representing the fold change relative to that of controls, which was converted to 1. For each gene (n=4; 2 values per embryo from 4 mutants), the mean values in the mutants were 0.07, 0.24 and 0.36 forEts2,Bmp4andNodal, respectively. The s.e.m. is shown by error bars (black lines) and all mutant values represent statistically significant fold changes (P<0.001), using the one-tailed unpaired Student’st-test. Full size image Figure 8:  Real-time PCR (qRT–PCR) gene expression level quantification in E6.7 Ets2 type-II mutant embryos. Graph showing the mean values of fold change for Ets2 , Bmp4 and Nodal mRNA levels in E6.7 mutants (dark grey columns) relative to those of E6.7 wild-type (wt) control embryos (light-grey columns). Both control and mutant values were relative to those of the internal control gene beta-actin , with mutant values representing the fold change relative to that of controls, which was converted to 1. For each gene ( n =4; 2 values per embryo from 4 mutants), the mean values in the mutants were 0.07, 0.24 and 0.36 for Ets2 , Bmp4 and Nodal , respectively. The s.e.m. is shown by error bars (black lines) and all mutant values represent statistically significant fold changes ( P <0.001), using the one-tailed unpaired Student’s t -test. Full size image To explore epiblast genes that could be upstream of Nodal and Snail , we first examined the expression of the transcription factor Foxh1 , which is required in the epiblast for maintaining Nodal expression levels [34] , [35] . Foxh1 expression in the epiblast of E6.7 mutants appeared normal ( n =4; Fig. 7g ), suggesting that it is not involved in regulating Nodal expression in this context. We subsequently investigated the expression of the secreted molecule Wnt3 , as it maintains epiblast Nodal expression levels in a largely Foxh1-independent fashion [36] , promotes mesoderm EMT by upregulating Snail expression [37] and is required in the epiblast for gastrulation processes that are strikingly similar to those affected in type-II mutants [38] . Wnt3 expression in E6.7 mutants is absent ( n =4; Fig. 7h ). To investigate whether the downregulation of Nodal and Wnt3 expression observed in E6.7 mutants is also evident at pregastrulation stages, we examined their expression at E6.4 and E6.3, respectively. Strikingly, both Nodal ( n =4) and Wnt3 ( n =3) are expressed at apparently normal levels in E6.3/6.4 mutants ( Fig. 7n–p ). Trophoblast gene expression in type-II mutants To explore how trophoblast Ets2 mediates gastrulation progression, we first examined the expression of the secreted molecule Bmp4, which is expressed specifically in the EXE before and during early gastrulation and can maintain epiblast Wnt3 expression [36] . EXE Bmp4 expression is extensively diminished in E6.7 mutants, based on RNA in situ hybridization ( n =3; Fig. 7k ) or qRT–PCR ( n =4; Fig. 8 ) and absent or abnormally low in E7.5–7.75 mutants ( n =3; Fig. 3d ). Previous experiments using trophoblast stem (TS) cells, the in vitro equivalent of EXE, showed that Ets2 is required for TS cell self-renewal and for maintaining the expression of several genes including Bmp4 , Cdx2 , Eomes , Esrrb and Pace4 [39] , [40] . The transcription factors Cdx2 and Elf5 are also required in TS cells for their self-renewal, with Cdx2 also maintaining Bmp4 expression [5] , [41] , [42] , [43] . We therefore examined the expression of all these genes in the EXE of type-II mutants at E6.7 and E7.5–7.75 and found that it was downregulated. Specifically, Cdx2 expression was either undetectable ( n =1/3) or greatly reduced ( n =2/3) at E6.7 ( Fig. 7m ) and absent at E7.5–7.75 ( n =3; Fig. 3e ), Pace4 ( n =3) and Elf5 ( n =3) were not expressed at E6.7 ( Fig. 7j ), the expression of Eomes was either undetectable ( n =1/3) or extremely low (2/3) at E6.7 ( Fig. 7b ) or absent at E7.75 ( n =5; Fig. 7c ) and Esrrb expression at E6.7 was either absent ( n =1/3) or barely detectable ( n =2/3) ( Fig. 7i ). As type-II mutants apparently lack EXE character (including Elf5 and Bmp4 expression) from E6.7 onwards (this study), we investigated whether this is also the case at pregastrulation stages by examining Bmp4 and Elf5 expression. Our results show that both are expressed normally in the EXE of E6.3 mutants ( n =3; Fig. 7o ). We show for the first time that the transcription factor Ets2 is required in trophoblast for the mediation of fundamental gastrulation processes after PS initiation. These include correct gene expression within the newly formed PS, elongation of the PS, completion of mesoderm EMT so as to allow migration of mesodermal cells away from the PS to form the mesoderm layer and correct development of anterior PS derivatives (for example, completion of DE formation and the appearance/specification of the node). This work also demonstrates that trophoblast signalling is not only required for gastrulation initiation [3] , [4] , [5] , [6] , but also for gastrulation progression. The latter is defined here as all gastrulation process taking place between E6.5 (PS initiation stage) and E7.75 (the stage just prior to the period when the embryo begins somitogenesis). Previous studies showed that trophoblast signalling is also required for correct PS development during somite stages, based on a subset of Bmp4 −/− conceptuses that can develop up to the 20-somite stage. Gastrulation in these mutants proceeds normally during pre-somite stages, but by the early somite stage there is abnormal mesodermal cell accumulation at the posterior PS, no allantois and abnormal node morphology (the overall shape of the ventral surface of the node was flat rather than concave) [18] , [44] . Chimaera analysis of this subset showed that Bmp4 is needed in EXE (or its derivative, the chorionic ectoderm) for correct posterior PS at the early somite stage, allantois formation and correct node morphology [17] , [18] , [44] . The lack of allantois could be caused by this late PS defect because the fate of posterior PS during late gastrulation is predominantly allantoic extraembryonic mesoderm [45] . It is not clear whether the node phenotype is due to defective gastrulation or due to intra-nodal processes occurring after node formation, as all node cell types were present in these mutants [18] , [44] . Interestingly, although a more severe subset of Bmp4 −/− conceptuses was reported to show ‘absence of an organized PS’ by E7.5 ( [17] ), suggesting a gastrulation progression defect, chimaera analysis of this subset to exclude a causative role for PS-derived Bmp4 ( Bmp4 is also expressed in the PS by E7.5) has not been done. How can the absence of Ets2 in trophoblast lead to the post-PS initiation gastrulation defects seen in Ets2 type-II mutants? We propose the following model that could explain this based on the data presented here and previous findings. Within the EXE, Ets2 maintains Bmp4 expression and EXE character (the in vivo equivalent of TS cell self-renewal) by directly maintaining the expression of Cdx2 , which directly conserves the expression of Bmp4 and that of the TS cell self-renewal transcription factor Elf5 , with Elf5 directly reinforcing Cdx2 expression. Subsequently, EXE-derived Bmp4 signalling from around E6.3-to-E6.7 onwards maintains epiblast Wnt3 expression, which in turn is responsible for two processes. The first is the maintenance of high epiblast Nodal expression levels for the mediation of PS elongation and anterior PS derivative development. The second is the induction of Snail expression in the PS for completion of mesoderm EMT to allow mesoderm migration. This model is supported by the following: (a) The trophoblast of Ets2 type-II mutants shows absence/reduction in the expression of Bmp4 , Cdx2 and Elf5 and that of other EXE character genes, such as Eomes , Esrrb and Pace4 , from around E6.7 onwards (this study). (b) Ets2 in TS cells is required for their self-renewal by maintaining the expression of Cdx2 ( [39] , [40] ), through direct binding to its promoter [39] , but not to those of Bmp4 , Eomes or Elf5 ( [46] ). (c) Cdx2 is required for TS cell self-renewal [42] and maintains the expression of Bmp4 ( [41] ) and Elf5 ( [42] ) by binding to their promoters in these cells [41] , [43] . (d) Elf5 in TS cells is needed for their self-renewal [5] and for the maintenance of Cdx2 and Eomes expression, through direct activation of their promoters [43] . (e) Bmp4, but not Nodal, is sufficient for maintaining Wnt3 expression in epiblast explants [36] . (f) Wnt3 maintains epiblast Nodal expression levels in a largely Foxh1-independent fashion [36] , promotes mesoderm EMT by upregulating Snail expression [37] and is required in the epiblast (but not VE) for gastrulation processes that take place after PS initiation and which are strikingly similar to those affected in type-II mutants, including PS elongation, intraembryonic mesoderm migration, node and AME formation, and completion of DE formation [38] . (g) High levels of epiblast Nodal expression/signalling are required for PS elongation and formation of anterior PS derivatives [9] , [30] , [31] . (h) Wnt3 and Snail expression levels are undetectable in the epiblast of E6.7 type-II mutants, while those of Nodal are greatly reduced (this study). The findings presented here suggest that Ets2-mediated trophoblast signalling for gastrulation progression after PS initiation is required between E6.3 and E6.7 because EXE character (marked by Elf5 expression) and EXE Bmp4 expression are lost from type-II mutants during this period, concomitant with the downregulation of Nodal and Wnt3 expression in their epiblast. These findings taken together with the observation that EXE ablation at E5.5, but not at E6.0, results in absence of PS formation [4] , may explain why type-II mutants initiate a PS, whereas type-I ones do not. That is, on Ets2 gene knockout, some mutants fail to initiate a PS because they lose EXE character/ Bmp4 expression from at least E5.5 (type-I phenotype) [4] , whereas other mutants initiate a PS (type-II phenotype) because they lose EXE character/ Bmp4 expression later, between E6.3 and E6.7 (this study). Developmental delay cannot be excluded as a cause for at least some of the defects observed in type-II mutants, as shown by the delayed onset of Eomes expression in the PS. Regarding the AVE anteriorization defect observed in the majority of type-II mutants, it is not clear whether the anterior edge of AVE never reaches the embryonic–extraembryonic junction or does so, but by E6.7 fails to maintain its localization. Interestingly, our failure to detect Foxh1 expression in the VE of type-II mutants could be related to this AVE defect, as Foxh1 is required in the VE, but not the epiblast, for correct positioning of the AVE [34] . However, further studies are needed to explore these issues. Embryo collection and genotyping Mice heterozygous for a null mutation of the Ets2 gene ( Ets2 db1 allele (ref. 7 )) were maintained on an outbred ICR (Institute of Cancer Research) genetic background [4] under standard housing conditions with the dark period of the light–dark cycle being between 20:00 and 6:00. These heterozygous mice were intercrossed to obtain homozygous Ets2 null conceptuses. Stage E0.5 was at 13.00 of the day a copulation plug was detected. Ets2 −/− conceptuses could be identified during dissection due to their relatively small size, reduced maternal blood accumulation around the conceptus and a V-shaped attachment of the Richert’s membrane at the distal tip of the embryo [4] , [7] . About half of Ets2 −/− mutants displayed the type-II phenotype, and the rest the type-I phenotype, as shown previously [4] . Type-II mutants could be distinguished morphologically from type-I ones based on several criteria, including the presence of a thickening of VE at the distal tip of the embryo and the absence of PS and mesoderm in the latter, as shown before [4] . Embryo genotype was confirmed by PCR of genomic DNA derived from either Richert’s membrane or proximal extraembryonic region or from the entire embryo after whole-mount in situ hybridization. Briefly, two separate PCR reactions were performed with a primer set that amplified either the wild-type (220 bp) or mutant (200 bp) allele. For the detection of the wild-type allele, the primers used were: 5′-CGTCCCTACTGGATGACAGCGG-3′ and 5′-TGCTTTGGTCAAATAGGAGCCACTG-3′. Those of the mutant allele were: 5′-CGTCCCTACTGGATGACAGCGG-3′ and 5′-AATGACAAGACGCTGGGCGG-3′. Both PCR reactions were carried out under the following conditions: 94 °C for 3 min; 35 × (94 °C for 30 s; 64 °C for 30 s; 74 °C for 4 s); 72 °C for 5 min. Whole-mount in situ hybridization Single-colour whole-mount in situ hybridization (either with one probe or two probes simultaneously) or double-colour whole-mount in situ hybridization (with two or three probes simultaneously) was carried out as previously described [4] . The plasmids for making riboprobes used for the detection of Bra , Nodal , Hex , Cer1 , Bmp4 , Foxh1 , Cdx2 , Cripto , Wnt3, Elf5, Pace4 and Esrrb expression have been described before [4] . Those for the detection of Chrd, Noto, Shh, Eomes, Gsc, Snail and Foxa2 were kindly provided by Dr Janet Rossant. Those for Fgf8 and Afp were kindly provided by Dr Tristan Rodriguez and Dr Anna-Katerina Hadjantonakis, respectively. Embryos were documented using an inverted microscope (Zeiss Axiovert 200M with AxioVision software). Histology Histology after whole-mount in situ hybridization was performed as before [4] . Briefly, embryos were post-fixed in 4% paraformaldehyde, dehydrated through an ethanol series and embedded in paraffin before sectioning (7-μm thickness). Semithin sections (1 μm-thick) were produced as described previously [4] from embryos fixed in 4% paraformaldehyde. Sections were visualized and documented using an inverted microscope (Zeiss Axiovert 200M with AxioVision software). Fluorescent immunohistochemistry Preparation of sections was done as described previously [47] . Briefly, embryos were fixed in 4% paraformaldehyde, dehydrated, embedded in paraffin wax and 7-μm-thick sections were cut using standard protocols. Deparaffinized sections underwent antigen retrieval (microwave heat treatment with TriSodium Citrate, pH 6, for 10 min). For detection of E-cadherin protein, sections were incubated with a primary rabbit anti-E-cadherin antibody (Abcam, ab53033) at 1:100 dilution, followed by incubation with an anti-rabbit IgG secondary antibody conjugated to Cy3 (Abcam, ab6939) at 1:100 dilution. Sections were then counterstained with Hoechst (nuclear marker). Finally, the sections were inspected and documented under fluorescence using a Zeiss Axio Imager.Z2 confocal microscope and zen 2010 software. Whole-mount DBA lectin histochemistry Fixed embryos in 4% paraformaldehyde at 4 °C either after fresh isolation or after whole-mount RNA in situ hybridization were at first washed in PBS/0.1% Triton-X100 and permiabilized in PBS/0.25% Triton-X100 for 30 min at room temperature, followed by wash in PBS/0.1% Triton-X100 for 10 min at room temperature. The embryos were then blocked for 1 h at room temperature with blocking solution (1% BSA, 0.1% Triton-X100, 10% goat serum in PBS) and incubated with biotinylated DBA lectin (L6533, Sigma) in blocking solution (without 0.1% Triton-X100) overnight at 4 °C (DBA dilution 1:3,000). This was followed by PBS/0.1% Triton-X100 washes at room temperature. They were then incubated with Streptavidin Peroxidase (Abcam, ab64269) for 15 min at room temperature and washed in PBS/0.1% Triton-X100. The desired colour was achieved by incubation in DAB (Abcam, ab64238), giving a brown signal, followed by PBS washes to stop the reaction. Embryos were visualized and documented using an inverted microscope (Zeiss Axiovert 200M with AxioVision software). qRT–PCR and statistical analysis Total RNA was isolated from individual E6.7 embryos (wild-type littermates and type-II mutants) using the ‘NucleoSpin RNA XS’ kit (Macherey-Nagel) according to the manufacturer’s instructions. Ten nanograms of RNA per embryo were reverse transcribed to generate complementary DNA, using reverse transcriptase (AMV, Finnzymes- Thermo Scientific) according to the manufacturer. qRT–PCR was performed using a Real-time thermal cycler CFX96 (Bio-Rad) with SYBR Green Power master mix (Applied Biosystems). The primers used were those for the Beta-actin gene (internal control), Ets2, Bmp4 and Nodal and were designed using the ‘Primer 3 Output’ software from cDNA sequences found in the NCBI Gene Database (Nucleotide). Their specificity was confirmed using a BLAST analysis against the genomic NCBI database. The primers were as follows: Beta-actin forward primer 5′-GACGGCCAGGTCATCACTAT-3′, Beta-actin reverse primer 5′-AAGGAAGGCTGGAAAAGAGC-3′ (product size, 68 bp); Ets2 forward primer 5′-GGGAGTTCAAGCTTGCTGAC-3′, Ets2 reverse primer 5′-CCCGAAGTCTTGTGGATGAT-3′ (product size, 139 bp); Nodal forward primer 5′-ACTTTGCTTTGGGAAGCTGA-3′, Nodal reverse primer 5′-ACCTGGAACTTGACCCTCCT-3′ (product size, 140 bp); Bmp4 forward primer 5′-CGTTACCTCAAGGGAGTGGA-3′, Bmp4 reverse primer 5′-ATGCTTGGGACTACGTTTGG-3′ (product size, 116 bp). qRT–PCR reaction conditions were: 50 °C for 2 min; 95 °C for 12 min; 39 × (95 °C for 20 s; 59 °C for 1 min; 72 °C for 30 s); 72 °C for 10 min. The relative quantification of gene expression between the mutants and control embryos was calculated by the 2 −ΔΔCt approximation method [48] . Two values per gene from four separate mutant embryos (that is, n =4) were obtained to calculate the mean +/− s.e.m. Statistical analysis was carried out using the one-tailed unpaired Student’s t -test. Differences were considered statistically significant for those with P <0.001. Generation of chimaeric conceptuses Chimaeras were generated as previously described [4] . Briefly, wild-type 129S6/B6-F1 hybrid ES cells ubiquitously expressing GFP were aggregated with tetraploid embryos (one tetraploid embryo per ES cell clump), and subsequently transferred to ICR recipients. The tetraploid embryos were produced from two-cell-stage embryos derived from crosses between Ets 2 db1 / Ets2 + heterozygotes, followed by electrofusion. The chimaeras were collected at around E7.75, viewed and documented under fluorescent microscopy using a GFP filter (inverted Zeiss Axiovert 200M microscope with AxioVision software). Subsequently, they were processed to be used for genotyping (proximal extraembryonic region or Richert’s membrane), followed by either semithin section histology or whole-mount in situ hybridization, as described above. How to cite this article: Polydorou, C. & Georgiades, P. Ets2-dependent trophoblast signalling is required for gastrulation progression after primitive streak initiation. Nat. Commun. 4:1658 doi: 10.1038/ncomms2646 (2013).